Robust site-resolvable quantum gates in an optical lattice via inhomogeneous control The power of optical lattices for quantum simulation and computation is greatly enhanced when atoms at individual lattice sites can be accessed for measurement and control. Experiments routinely use high-resolution microscopy to obtain site-resolved images in real time, and site-resolved spin flips have been implemented using microwaves resonant with frequency-shifted target atoms in focused light fields. Here we show that methods adapted from inhomogeneous control can greatly increase the performance of such resonance addressing, allowing the targeting of arbitrary single-qubit quantum gates on selected sites with minimal cross-talk to neighbouring sites and significant robustness against uncertainty in the atom position. We further demonstrate the simultaneous implementation of different gates at adjacent sites with a single global microwave pulse. Coherence is verified through two-pulse experiments, and the average gate fidelity is measured to be 95±3%. Our approach may be useful in other contexts such as ion traps and nitrogen-vacancy centres in diamond. Ultracold atoms in optical lattices [1] are an important platform for quantum information science, lending itself naturally to quantum simulation of many-body physics [2] and providing a possible path towards a scalable quantum computer [3] , [4] . Quantum simulations with the atom-lattice system generally explore many-body physics of condensed matter systems described by simple model Hamiltonians, for example, the families of Hubbard [5] and Ising [6] models, and similar physics is typically relevant when exploring optical lattice-based architectures for universal quantum computing [7] , [8] . Thus, although optical lattices in principle can have spatial periods from one-quarter to many times the optical wavelength, the need for site-to-site tunnelling in such experiments tends to limit the workable lattice period to <1 μm. That in turn poses a significant obstacle to the implementation of reliable, high-fidelity quantum control of atoms at individual lattice sites, which will ultimately be required to reach the full potential of this system. Atoms in two-dimensional (2D) lattices with periods near the optical wavelength have been successfully imaged using high numerical aperture optics with resolution close to the lattice spacing [9] , [10] . Other demonstrations include cavity-aided magnetic resonance imaging [11] , optical microscopy in conjunction with numerical deconvolution [12] and imaging in a three-dimensional (3D) lattice with ∼ 5 μm period [13] . Coherent quantum control of atoms at targeted lattice sites requires even higher resolution than imaging if adjacent atoms are to remain unperturbed. Subwavelength resolution can in principle be achieved with a tightly focused optical field that shifts the transition frequency of an atomic qubit relative to its neighbours, in combination with a frequency selective microwave pulse that implements the desired rotation of the targeted qubit [14] . In practice, such a resonance-addressing scheme involves a tradeoff—for a sharply focused addressing field, the frequency shift becomes overly sensitive to its alignment relative to the target site, whereas a softer focus leads to unwanted perturbations at adjacent sites. Faced with these difficulties, experiments have so far demonstrated only adiabatic spin flips [15] , which are robust to small variations in the frequency shift but cannot manipulate coherence between the spin-up and spin-down states in the manner of universal quantum gates. Misalignment between the trapping and addressing fields can be avoided by incorporating a spatially varying qubit frequency shift into the lattice itself. This approach has been used to target quantum gates on sub-ensembles of qubits located on one or the other side of the barrier in a lattice consisting of double wells, but does not lend itself to more general forms of addressing [16] . In this article, we explore the use of advanced quantum control to dramatically improve and extend the capabilities of resonance addressing. It is known from the theory of inhomogeneous control in nuclear magnetic resonance that composite pulses can be designed to achieve any desired qubit response as a function of one or more parameters [17] , [18] , [19] . Applying this idea to resonance addressing, we first map position onto frequency shift and then design a single phase-modulated microwave pulse to implement a unitary transformation that is a chosen function of that frequency shift. An example might be a pulse that executes a quantum gate across a desired frequency and spatial interval, while at the same time doing nothing (the identity transformation) outside it. We show that such a ‘top-hat’ response can greatly improve the robustness against misalignment between trapping and addressing fields, while at the same time suppressing perturbation of the adjacent sites. We further show that it is possible to simultaneously perform different gates at adjacent sites with a single global control waveform. In both cases, we verify coherent gate operation through two-pulse Ramsey interrogation, and use randomized benchmarking [20] to measure an average gate fidelity of 95±3%. This control-based approach to reduce cross-talk and increase robustness is broadly applicable in optical lattices irrespective of geometry, and may be useful also on other platforms for quantum information processing, such as ion traps [21] and nitrogen-vacancy centres in diamond [22] . Preparing and imaging the atom sample To test the basic idea in the laboratory, we have implemented spatially resolved resonance addressing along one dimension of a 3D optical lattice with a Λ=426 nm period, using a superimposed optical standing wave—the ‘addressing lattice’—as illustrated in Fig. 1a . The trap lattice is loaded with caesium atoms at a density of one atom per ∼ 100 sites, each representing a qubit encoded in two spin states, and . The addressing lattice is formed by two laser beams intersecting at a shallow angle, producing a frequency shift that varies sinusoidally along the x axis of the trap lattice as shown in Fig. 1b . Because the frequency shift is uniform in the y–z plane, this geometry addresses ∼ 35 planes of ∼ 10 3 atoms simultaneously, rather than individual sites in the 3D trap lattice. 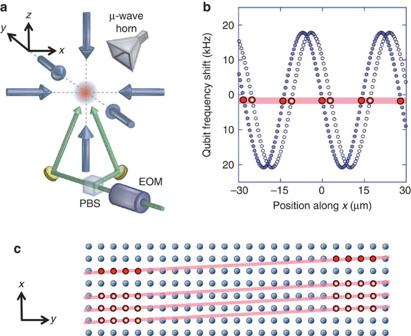Figure 1: Trapping and addressing in an optical lattice. (a) Atoms are trapped in a 3D lattice (blue), in the presence of a one-dimensional addressing lattice (green) that can be translated using an electro-optic modulator (EOM) and polarization beamsplitter (PBS). (b) Variation in the qubit transition frequency for sites in the trap lattice (blue dots). A narrow-band microwave pulse of appropriate frequency (red line) addresses atoms at resonant sites (red dots). Translation of the addressing lattice (blue circles) targets atoms at different sites (red circles). (c) Schematic of trap lattice sites in thex–yplane. A slight misalignment between the planes of the trap and addressing lattices ensures the presence of resonant sites (top red line and filled red circles) for any microwave frequency and position of the addressing lattice. Translating the addressing lattice alongxallows sequential addressing of adjacent sites (bottom red lines and open red circles), for example, triplets of sites separated by exactly one period of the trap lattice as shown here. Figure 1: Trapping and addressing in an optical lattice. ( a ) Atoms are trapped in a 3D lattice (blue), in the presence of a one-dimensional addressing lattice (green) that can be translated using an electro-optic modulator (EOM) and polarization beamsplitter (PBS). ( b ) Variation in the qubit transition frequency for sites in the trap lattice (blue dots). A narrow-band microwave pulse of appropriate frequency (red line) addresses atoms at resonant sites (red dots). Translation of the addressing lattice (blue circles) targets atoms at different sites (red circles). ( c ) Schematic of trap lattice sites in the x–y plane. A slight misalignment between the planes of the trap and addressing lattices ensures the presence of resonant sites (top red line and filled red circles) for any microwave frequency and position of the addressing lattice. Translating the addressing lattice along x allows sequential addressing of adjacent sites (bottom red lines and open red circles), for example, triplets of sites separated by exactly one period of the trap lattice as shown here. Full size image The addressing lattice is translated with nanometre accuracy along x by changing the relative optical phase between the addressing beams. Passive stability keeps jitter in the relative position of the trap and addressing lattices <15 nm on a timescale of several seconds, sufficient that it can be regarded as constant during a single run of the experiment, whereas on timescales from minutes to hours, the lattice positions may drift by several microns. For the purpose of our experiments here, the effects of this slow drift can be eliminated using a preparation and resonance imaging protocol described in the following. To prepare a well-defined starting point, we select a subset of atoms in the trap lattice, by flipping their spins from to with a narrow-band microwave pulse and removing the remaining atoms in . In this situation, the spin-flip probability depends on the qubit transition frequency and thus on the position of the atoms relative to the addressing lattice ( Fig. 1b ). By introducing a slight tilt between the planes of the trap and addressing lattices, we ensure that there will always be a subset of sites in the trap lattice whose resonance frequencies lie within the bandwidth of the ‘preparation pulse’, no matter the relative position of the lattices ( Fig. 1c ). The result is an ensemble of atoms prepared in the state at sites in the trap lattice that have a precisely controllable distribution of spatial offsets relative to the nominal target plane. We can construct a high-resolution resonance image of an atom distribution thus prepared, through repetitions of the experiment wherein the preparation step is followed by a translation of the addressing lattice, a second ‘imaging pulse’, and a measurement of the number of atoms returned to the state. 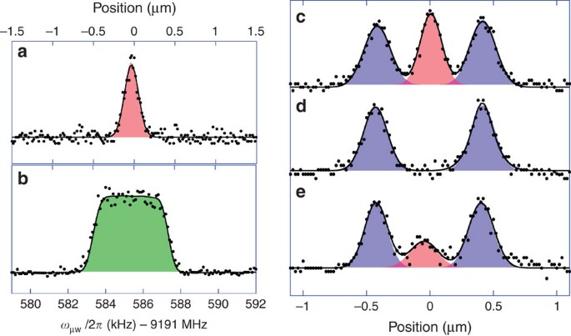Figure 2: Resonance imaging and addressing of single and multiple planes. (a) Resonance image showing a distribution of atoms prepared in a single plane as indicated inFig. 1c. (b) Spin-flip probability for a composite microwave pulse with a ‘top-hat’ response as function of frequency. The frequency and position axes are matched betweenaandb. (c) Preparation of atoms in three adjacent planes as inFig. 1c. (d) Selective spin flip of atoms at the centre sites, performed using a composite pulse with a top-hat response similar to, but narrower than,b. (e) Imperfect spin flip of atoms at the centre sites, performed using a Gaussian pulse. Solid dots represent data and lines represent fits. Inaandc–e, the shaded areas show the separate Gaussians fits associated with atoms at adjacent sites. Figure 2a shows such an image, together with a Gaussian fit with s.d. σ =80 nm. The image width is given by the convolution of the (identical) preparation and imaging pulses, and indicates a spatial resolution of ∼ 56 nm, well below the lattice period. It is also possible to prepare and image atom distributions in planes that are separated by, for example, one trap lattice period along x , by applying a sequence of preparation pulses with identical frequency and separated by appropriate translations of the addressing lattice ( Fig. 1c ). A resonance image of an atom distribution corresponding to triplets of adjacent sites along x is shown in Fig. 2c . Figure 2: Resonance imaging and addressing of single and multiple planes. ( a ) Resonance image showing a distribution of atoms prepared in a single plane as indicated in Fig. 1c . ( b ) Spin-flip probability for a composite microwave pulse with a ‘top-hat’ response as function of frequency. The frequency and position axes are matched between a and b . ( c ) Preparation of atoms in three adjacent planes as in Fig. 1c . ( d ) Selective spin flip of atoms at the centre sites, performed using a composite pulse with a top-hat response similar to, but narrower than, b . ( e ) Imperfect spin flip of atoms at the centre sites, performed using a Gaussian pulse. Solid dots represent data and lines represent fits. In a and c – e , the shaded areas show the separate Gaussians fits associated with atoms at adjacent sites. Full size image Spin flips and quantum gates Robust control in the presence of broad distributions of qubit positions and frequencies requires the use of more advanced techniques such as phase-modulated microwave pulses. These composite pulses consist of a train of N square pulses with variable phases { φ j } that have been computer optimized, so that the overall transformation accomplishes a desired objective [17] , [18] . This can be either a spin rotation on a fixed input state, , or a full unitary transformation (quantum gate) W ( δ ) that varies in a prescribed way with the frequency shift δ of the qubit resonance relative to the microwave frequency (see Methods). Figure 2b shows the response to a composite pulse designed to flip spins uniformly across a targeted frequency region and leave them unaffected elsewhere. We can test the performance of a similar top-hat pulse whose three regions have been optimized to overlap with an atom distribution corresponding to triplets of adjacent sites. Figure 2d shows the distribution after the pulse, indicating a complete, robust spin flip at the centre sites, and a complete, robust absence of spin flips at the adjacent sites. For comparison, Fig. 2e shows the result of applying a single Gaussian pulse (identical to the preparation pulses) resonant at the centre of the distribution. In this case, some spins at the centre sites are unaffected, whereas some spins at the adjacent sites have been flipped. Adjusting the width of the pulse allows a tradeoff between the two types of error, but performance never approaches that of Fig. 2d . The performance of unitary quantum gates can be evaluated with a two-pulse version of the approach above. We begin by applying a composite pulse that implements a π /2 rotation around the i axis of the Bloch sphere in the central frequency region and the identity elsewhere. Shifting the overall phase of the pulse by φ changes the axis of rotation to cos( φ ) i +sin( φ ) j , and two pulses in sequence lead to a spin-flip probability cos 2 ( φ /2), similar to the φ -dependent interference in a two-path interferometer. 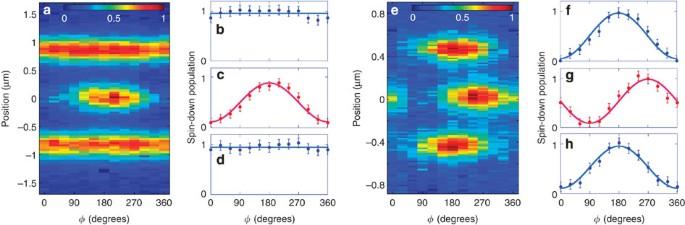Figure 3: Unitary quantum gates. (a) Sequence of colour-coded resonance images (similar toFig. 2c), showing the coherent action of a pair of composite pulses. Each pulse implements aπ/2 rotation on the central atom distribution, with full spin flips occurring atφ=0° and 360°, and the identity atφ=180°. Both the individual pulses and the pair always implement the identity on the adjacent atom distributions. (b–d) Population remaining in the initialstate as function of relative pulse phase, for each distribution. The populations (dots) are determined from the areas of Gaussian fits as inFig. 2c. Solid lines are fits to the interference pattern, and error bars are estimated as 1 s.d. of the residuals from the fit. (e–h) Sequence of resonance images and interference patterns similar toa–d, but with atom distributions chosen to coincide with adjacent sites alongx. The first composite pulse here implements a Hadamard pulse at the centre sites and aπ/2 rotation at the adjacent sites, and the second pulse implementsπ/2 rotations at every site. Solid lines are fits to the interference pattern, and error bars are estimated as 1 s.d. of the residuals from the fit. Figure 3a–d shows a sequence of resonance images and corresponding populations remaining in as a function of the phase φ . The clear interference for atoms in the central region and the lack of φ dependence for atoms in the adjacent regions demonstrate that the pulse functions as intended and coherence is preserved. Figure 3: Unitary quantum gates. ( a ) Sequence of colour-coded resonance images (similar to Fig. 2c ), showing the coherent action of a pair of composite pulses. Each pulse implements a π /2 rotation on the central atom distribution, with full spin flips occurring at φ= 0° and 360°, and the identity at φ= 180°. Both the individual pulses and the pair always implement the identity on the adjacent atom distributions. ( b – d ) Population remaining in the initial state as function of relative pulse phase, for each distribution. The populations (dots) are determined from the areas of Gaussian fits as in Fig. 2c . Solid lines are fits to the interference pattern, and error bars are estimated as 1 s.d. of the residuals from the fit. ( e – h ) Sequence of resonance images and interference patterns similar to a – d , but with atom distributions chosen to coincide with adjacent sites along x . The first composite pulse here implements a Hadamard pulse at the centre sites and a π /2 rotation at the adjacent sites, and the second pulse implements π /2 rotations at every site. Solid lines are fits to the interference pattern, and error bars are estimated as 1 s.d. of the residuals from the fit. Full size image A second example of a two-pulse experiment is shown in Fig. 3e–h ; in this case, for frequency regions that correspond to triplets of adjacent sites as in Fig. 2c . Here the first pulse implements a Hadamard gate (rotation by π around the axis) on the centre sites and π /2 rotations on the adjacent sites. The second pulse implements identical π /2 rotations at every site, leading to interference patterns similar to Fig. 3c but with a 90° shift at the centre sites. This data set shows explicitly that the gate operations are coherent on every site, and also demonstrates the freedom to perform independent gates simultaneously at adjacent sites with a single composite pulse. The contrast of the interference patterns in Fig. 3f–h provides information about the fidelity of the various transformations. We can estimate the overall fidelity of a two-gate sequence as pair = S ma x /( S min + S max ), where S min and S max are the minimum and maximum values of the interference signal. Assuming that gate errors are small, ɛ =1−<<1, uncorrelated, and independent of φ , the gate fidelity can then be estimated as . For the data in Fig. 3f–h , this yields an average gate fidelity of =0.96. Randomized benchmarking A more comprehensive test of gate fidelity is best performed using randomized benchmarking [20] . This approach separates gate errors from errors in the preparation of input states and measurement of output states, and provides a meaningful measure of the average fidelity of gates when they are combined into long random sequences. For the 4 ms pulses used in Fig. 3 , the total duration of the necessary pulse sequences exceeds the time available in our experiment, but useful information can still be obtained by benchmarking a set of pulses that have been rescaled and shortened to 1 ms duration in such a way that the intrinsic control fidelity remains unchanged (see Methods). 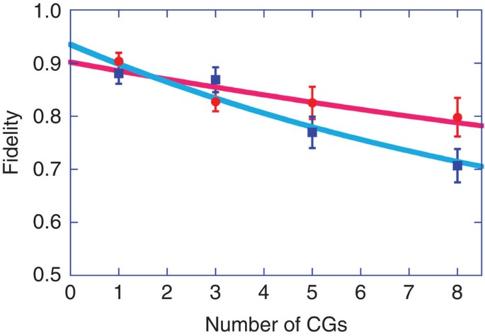Figure 4: Randomized benchmarking. Overall fidelities achieved by sequences of composite pulses that apply computational gates (CGs) and Pauli randomizing gates (PGs) to the central atom distribution (red), and repeated identities to the adjacent ones (blue). Dots and squares are experimental data and lines are fits. Error bars are 1 s.d., estimated from the spread of fidelities seen in different sequences. Figure 4 shows the fidelity for sequences of rescaled pulses that were originally designed to implement computational gates (CGs) on the target lattice sites and the identity at neighbouring sites. Fits yield an average fidelity CG =0.98 for the central region, and a fidelity per identity of I =0.96 for the adjacent regions. In the absence of external perturbations, for example, magnetic fields and light scattering, one would expect similar fidelities for the site-resolvable gates implemented by the original pulse. On the other hand, if gate errors were entirely due to external factors, one might expect four times the error for the original pulses. This implies a fidelity in the range CG =0.92−0.98 for the site-resolvable quantum gates in Fig. 3 . This is consistent with the ∼ 0.96 obtained from the two-pulse interference patterns, especially because the latter estimate includes a non-negligible contribution from initialization and readout errors. Figure 4: Randomized benchmarking. Overall fidelities achieved by sequences of composite pulses that apply computational gates (CGs) and Pauli randomizing gates (PGs) to the central atom distribution (red), and repeated identities to the adjacent ones (blue). Dots and squares are experimental data and lines are fits. Error bars are 1 s.d., estimated from the spread of fidelities seen in different sequences. Full size image Our laboratory realization of robust, site-resolvable quantum gates through quantum control points to further experiments aimed at control of atoms in optical lattices. In our geometry, increasing the gradient of the frequency shift will allow the implementation of faster quantum gates with shorter pulses, while increasing the pulse amplitude and number of phase steps will allow the simultaneous implementation of independent gates across a much larger number of lattice sites and reduce the overhead associated with serial resonance addressing. Most importantly, the use of a focused addressing field [15] should make it straightforward to address a single site in a 2D or 3D optical lattice. From a control perspective, this task is simpler than the one undertaken here, because one only has to consider the atomic response in two regions—one covering frequency shifts near the focus, and one covering the remaining range of frequency shifts down to zero. Further developments might use site-resolved single-atom control to ‘activate’ [8] qubits for detection, or for the implementation of localized two-qubit gates through cold collisions or dipole–dipole interactions between Rydberg atoms [23] , [24] . Ultimately, the ability to simultaneously execute quantum logic gates on different qubits could substantially reduce the computational time complexity of quantum algorithms. With such parallelization, the circuits for the Quantum Fourier Transform and encoding/decoding of quantum-error correcting codes with O ( n ) qubits can be compressed to O (log n ) operations [25] , [26] . Other paradigms such as measurement-based quantum computation also benefit from parallelization; almost all gates can be implemented simultaneously in a single control and measurement step [27] . Atom trapping and manipulation Our trap lattice is formed by three pairs of counter propagating laser beams with parallel linear polarizations, tuned 140 GHz above the 6 S 1/2 ( f =4)→6 P 3/2 ( f ′ =5) hyperfine transition at 852 nm. The depth of the optical potential is ∼ 40 μK, corresponding to a trap vibrational frequency of 20 kHz. We load the trap lattice with 10 7 atoms from a magneto-optic trap and optical molasses, with a density of one atom per 100 sites in a volume with a diameter of ∼ 35 addressing lattice periods. Qubits are encoded in states and in the hyperfine ground state. We use sideband cooling [28] , [29] , [30] to prepare atoms in the state, with mean vibrational excitation ≈0.01 along x (excitation along y and z is unimportant). A bias magnetic field separates the qubit transition frequency from others in the ground manifold, and the combined bias, DC and AC background magnetic fields are stabilized to better than 20 μG using an approach similar to Smith et al. [31] The resulting frequency variation in the qubit transition frequency is ∼ 50 H z . The atomic qubits are driven with 9.2 GHz microwaves from two horn antennae adjusted to improve the field homogeneity across the atom cloud. Selective removal of atoms in the state is accomplished with radiation pressure from a resonant laser beam. Populations of the and states are obtained via Stern–Gerlach measurement. Addressing lattice The addressing lattice is formed by two plane waves with orthogonal linear polarizations, intersecting at an angle of 1.74°. This configuration creates a lattice of constant intensity and spatially varying polarization. The corresponding light shift is equivalent to a fictitious magnetic field [32] , with the steepest gradient where its value is near zero ( Fig. 1b ), the most favourable situation for resonance imaging and addressing. The addressing lattice period is 28 μm, corresponding to 65.9 periods of the trapping lattice. For perfectly aligned trap and addressing lattices, such incommensurate periods would slightly shift the relative position of the trap sites from period to period of the addressing lattice, but this becomes irrelevant for misaligned lattices as discussed in the main text. Calibrating translations and frequency shifts The addressing lattice is translated along x by shifting the relative phase between its plane wave components with an electro-optic modulator (EOM) in the beam path ( Fig. 1a ). To prepare atoms in adjacent planes ( Fig. 1c ), an accurate calibration of translation as a function of the EOM control voltage is required. This calibration is performed by preparing atoms in a single y–z plane at position x 0 , displacing them a known distance Δ x along x , constructing a resonance image and noting the EOM voltage at the image centre where the addressing lattice has been translated by the same Δ x . As illustrated in Supplementary Fig. S1a , atoms are moved by changing the angle θ between the linear polarizations of the beams making up the trap lattice along x , with angles θ ={−360°,−180°, 0°, 180°, 360°} resulting in displacements Δ x ={−Λ,−Λ/2, 0, Λ/2, Λ}, where Λ=426 nm is the trap lattice period [33] . Supplementary Figure S1b shows resonance images for various polarization angles θ . A fit to the EOM voltages at the image centres ( Supplementary Fig. S1c ) shows an addressing lattice translation of one trap lattice period per 164 V, consistent with independent measurements of the EOM phase shift and the intersection angle of 1.74° between the addressing lattice beams. Once the translation versus EOM voltage is known, the spatial gradient of the frequency shift in the addressing lattice can be determined. This is done by preparing atoms in a single plane near the point of steepest gradient, applying a known Zeeman shift Δ ω of the qubit transition frequency with an external magnetic field ( Supplementary Fig. S2a ), and constructing a resonance image ( Supplementary Fig. S2b,c ). Because atoms are trapped at points of positive as well as negative gradient, a frequency shift Δ ω ≠0 produces a double-peaked resonance image. An accurate measure of the frequency shift gradient can then be obtained from the peak separations versus Zeeman shift ( Supplementary Fig. S2d ). Microwave pulse design Atom preparation and resonance imaging are performed with microwave pulses having fixed frequency and phase, and a Gaussian envelope with a s.d. of 0.5 ms in the time domain. The corresponding power spectrum is also Gaussian with a root mean square width of 225 Hz. More advanced control is performed with composite microwave pulses consisting of a train of N square pulses having common amplitude A , duration T and frequency , but with phases ϕ j that vary between each pulse in the train. We keep fixed and use the set of phases { ϕ j }, along with A , T and the detuning δ = ω qubit − ω μw from qubit resonance, as our control parameters. Each of the square pulses has Rabi frequency Ω 0 ∝ A , duration T , detuning δ and a phase ϕ j , and will implement a unitary transformation U ( ϕ j , A , T , δ )=exp[− i ( θ /2) · q j ] that corresponds to a rotation of the qubit Bloch vector by an angle θ = Ω T around an axis q j =( Ω 0 / Ω )cos( ϕ j ) i +( Ω 0 / Ω )sin( ϕ j ) j +( δ / Ω ) k , where is the generalized Rabi frequency, and ={ σ i , σ j , σ k } is the vector of Pauli operators. In that case, the composite rotation implemented by all N pulses is an overall transformation . We can then use standard numerical techniques to search for control parameters that achieve a desired objective, for example, implementing a quantum logic gate W ( δ ) that is a prescribed function of δ . This is done by defining a cost function; in our case, the distance between the target and actual unitary matrices, averaged over a frequency band Δ, where is the Hilbert–Schmidt distance between W and U . Minimizing C then finds a set of values { ϕ j }, A , T such that U N ({ ϕ j }, A , T , δ )≈ W ( δ ). Note that this cost function includes the overall phase between U and W ; because this phase is not physically meaningful, the control task could be simplified by instead maximizing the frequency average of |Tr( U † W )|. Different control objectives can be achieved by substituting an appropriate cost function, for example, for frequency-dependent spin flips, the cost function is the infidelity averaged over the relevant frequency interval, , where is the desired final spin state as function of δ . Numerical searches for controls { ϕ j }, A , T that minimizes a given cost function are performed in Matlab, using any of several unconstrained non-linear optimization routines from the standard library. Design of a single control waveform takes an average of 8 h on a laptop computer, but the process can be speeded up significantly by using an advanced search algorithm such as GRAPE [34] , and by running a number of independent searches in parallel on different processors in a cluster. Microwave source We use an inexpensive microwave source as depicted in Supplementary Fig. S3a , combining an HP8672A Synthesized Signal Generator, which supplies a carrier at 9.2 GHz, and a Tabor WW2572A-2 Direct Digital Synthesis Arbitrary Waveform Generator, which supplies a signal at 30 MHz. The two are mixed in a single-sideband mixer whose output is preamplified, split in two, passed through a pair of 2 W power amplifiers and radiated by a pair of horn antennae with 15 dB gain. A low-power microwave switch between the HP8672A and the mixer is used for digital on/off control, whereas amplitude, frequency and phase modulation of the WW2572A-2 under internal arbitrary waveform control is used to correspondingly modulate the sideband used to drive the atomic qubits. The overall system delivers microwave fields with amplitude sufficient to drive the qubit transition with Rabi frequencies up to 40 kHz. The amplitude-modulation capability is used when we generate preparation and imaging pulses with Gaussian envelope in the time domain, whereas the phase-modulation capability is used when we generate composite pulses for more advanced inhomogeneous control. An example of the time-dependent qubit Rabi frequency (proportional to μw amplitude) and phase of one of these composite pulses is shown in Supplementary Fig. S3b,c . Pulse rescaling As stated above, the j th square pulse in a pulse train rotates the qubit Bloch vector by an angle θ = Ω T around an axis q j . It follows that replacing Ω 0 → κ Ω 0 , T → T / κ and δ → κδ leaves the angle and axis of rotation unchanged. Extending this to an entire pulse train, we see that U N ({ ϕ j }, A , T , δ )= U N ({ ϕ j }, κA , T / κ , κδ ). This implies that if a pulse train implements U N ({ ϕ j }, A , T , δ )≈ W ( δ ), then a rescaled pulse train implements U N ({ ϕ j }, κA , T / κ , δ )≈ W ( δ / κ ), with the same value of the cost function when averaged over a bandwidth κ Ω . As a result, a composite pulse can be rescaled to stretch or compress it in the time domain while compressing or stretching it in the frequency domain, without otherwise changing the fidelity with which it implements the desired objective (the intrinsic control fidelity). Randomized benchmarking Following Knill et al. [20] , we perform randomized benchmarking by initializing atoms in the state, applying l successive pairs of π /2 CGs and PGs, and reading out the overall fidelity with which the qubit is returned to the state. The sequence is repeated with random choices of CGs and PGs to obtain average overall fidelities as function of l . This data is then fitted with a function F ( l )=[1+(1− ɛ 0 )(1−2 ɛ ) l ]/2, where ɛ 0 is the combined initialization and readout error, and ɛ is the average error per CG. To fit a sufficient number of composite pulses into the time window available in the experiment, we shorten them to 1 ms (rescaling by κ =4). Provided that errors are dominated by imperfections in the control fields, and that the pulses are tested on a broadened version of the distribution in Fig. 2c , benchmarking will then provide a valid measure of the experimental gate fidelity. How to cite this article: Lee, J. H. et al. Robust site-resolvable quantum gates in an optical lattice via inhomogeneous control. Nat. Commun. 4:2027 doi: 10.1038/ncomms3027 (2013).